Controlling spins in adsorbed molecules by a chemical switch The development of chemical systems with switchable molecular spins could lead to the architecture of materials with controllable magnetic or spintronic properties. Here, we present conclusive evidence that the spin of an organometallic molecule coupled to a ferromagnetic substrate can be switched between magnetic off and on states by a chemical stimulus. This is achieved by nitric oxide (NO) functioning as an axial ligand of cobalt(II)tetraphenylporphyrin (CoTPP) ferromagnetically coupled to nickel thin-film (Ni(001)). On NO addition, the coordination sphere of Co 2+ is modified and a NO–CoTPP nitrosyl complex is formed, which corresponds to an off state of the Co spin. Thermal dissociation of NO from the nitrosyl complex restores the on state of the Co spin. The NO-induced reversible off–on switching of surface-adsorbed molecular spins observed here is attributed to a spin trans effect. Planar organometallic complexes with extended π -conjugation, for example, metalloporphyrins and metallophthalocyanines, have an indispensable role in controlling a wide range of functionalities: chemical reactivity (in biochemistry), optical absorbance (in dyes), optoelectronic conductance (in light harvesting chromophores), as well as the ability to function as electron donors or acceptors (in gas sensors and organic semiconductor devices) [1] . This degree of control is achieved by modifying the coordination of the central metal ion through interaction with its environment, for example, by an external chemical stimulus, as exemplified in nature by the regulation of Fe-porphyrin-to-oxygen affinity within the haemoglobin tetramer [2] , [3] . Recently, a similar effect has been implemented at surfaces in which the electronic surface-molecular interaction has been controlled by chemical stimuli [4] , [5] , [6] . Furthermore, metalloporphyrins containing unpaired spins have been shown to exhibit exchange coupling to magnetic substrates [7] , [8] , [9] , [10] , [11] , [12] . In view of spintronics [13] , [14] , which has been predominantly emerging for thin-film devices such as spin valves and transistors, it comprises a challenge to control single molecular spins within their specific environment at the spintronic interface. Notably, the molecular spin state for inorganic complexes/polymers in bulk can be controlled by external factors such as temperature, pressure and photon-induced excitation [15] , [16] , [17] , [18] . Molecules containing unpaired spins and molecular magnets bearing several coupled magnetic atoms [19] have recently received increasing attention. Unpaired electron spins in a molecule offer a wide range of options towards the tuning of their coupling with the environment. The structure and properties of such molecules can be initially architectured through synthesis and can be further modified by chemical reactions. X-ray magnetic circular dichroism (XMCD) spectroscopy [20] , [21] allows for the highly sensitive determination of the magnetization of spin systems assembled at surfaces with elemental and chemical specificity. The XMCD technique has also been used to assess the magnetization of adsorbed metalloporphyrin spin systems with respect to ferromagnetic substrates [7] , [8] , [9] , [10] , [11] . In this article, we demonstrate that the spin of a metalloporphyrin molecule, namely cobalt(II)tetraphenylporphyrin (CoTPP), is magnetically coupled to a ferromagnetic substrate (here nickel (Ni(001))) and can be controlled by nitric oxide (NO) functioning as a chemical stimulus. A reversible off–on switching process of the molecular spin, induced by NO, in the presence of the remanent magnetization of the Ni substrate is shown. Addition of NO supersedes the Co–Ni magnetoelectronic interaction by the formation of a NO–CoTPP nitrosyl complex [22] , [23] , which corresponds to the off state of the Co spin in CoTPP. Thermal dissociation of NO from the nitrosyl complex restores the initial Co–Ni magnetoelectronic interaction and leads to the on state of the Co spin in CoTPP. Thereby, this work provides an example of a chemical switch affecting the spin in surface-adsorbed molecules and presents a case for the spin trans effect in analogy to the well-established ' trans effect' [22] , [23] , [24] . Using stimuli to control single atomic [25] and molecular spins at interfaces and determining their coupling with the environment is of eminent interest in the field of quantum information [26] . Design of the magnetic interface A cobalt-porphyrin, CoTPP (see Fig. 1a ; top panel), has been chosen as a magnetic molecule characterized by one unpaired electron ( S =½; magnetic moment M (static)=1.73 μ B , M (effective)=1.92 μ B ) [27] . On the basis of its architecture and properties, this molecule is expected to be affected by the up or down magnetization of the ferromagnetic Ni substrate [8] . Atomically clean Ni substrates were prepared by deposition of thin films (~20 monolayers (MLs)) onto clean Cu(001) single crystals in ultrahigh vacuum. About 1 ML of CoTPP molecules was then evaporated onto the freshly prepared non-magnetized Ni(001) substrates kept at room temperature. On such prepared samples the magnetization of the different elemental species, that is, Co and Ni, has been determined by the element-specific XMCD technique [20] (see Fig. 1a ; bottom panel). 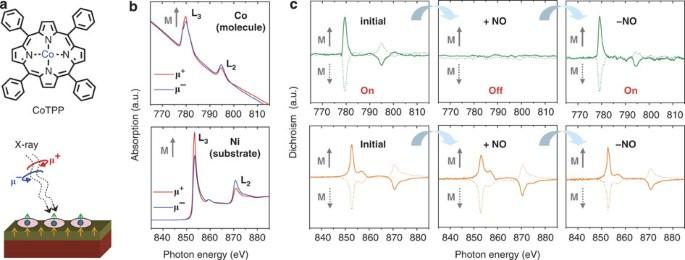Figure 1: Magnetic ordering of substrate (Ni) and organic adsorbate (CoTPP) with respect to the NO-induced switching. In all spectra, 'a.u.' represents arbitrary units. (a) Chemical structure of the CoTPP molecule (top) and schematic view of the XMCD experiment (bottom). (b) Chemical identification of Co and Ni: L-edges X-ray absorption spectra of Co (CoTPP, photon energy range: 765–815 eV) and Ni (substrate, photon energy range: 835–885 eV) acquired with circularly polarized X-ray light from a synchrotron source with opposite helicities (μ+and μ−). The difference in X-ray absorption for the opposite helicities (dichroism) reveals the magnetization of the observed chemical species. (c) Spin-switching sequence from left to right as indicated by arrows: L-edges XMCD spectra of Co (top panels) and Ni (bottom panels) recorded on the CoTPP/Ni(001) system after the initial preparation of molecular adlayers (left), after NO addition (centre) and on temperature-induced NO desorption (right). The directions of the remanent substrate magnetization M are indicated by grey arrows to the left of each spectrum. Ferromagnetic ordering of molecular spins with respect to the substrate is observed initially. Reversible 'off–on' switching of Co magnetization is observed with progressing NO addition and temperature-induced NO desorption. Figure 1: Magnetic ordering of substrate (Ni) and organic adsorbate (CoTPP) with respect to the NO-induced switching. In all spectra, 'a.u.' represents arbitrary units. ( a ) Chemical structure of the CoTPP molecule (top) and schematic view of the XMCD experiment (bottom). ( b ) Chemical identification of Co and Ni: L-edges X-ray absorption spectra of Co (CoTPP, photon energy range: 765–815 eV) and Ni (substrate, photon energy range: 835–885 eV) acquired with circularly polarized X-ray light from a synchrotron source with opposite helicities (μ + and μ − ). The difference in X-ray absorption for the opposite helicities (dichroism) reveals the magnetization of the observed chemical species. ( c ) Spin-switching sequence from left to right as indicated by arrows: L-edges XMCD spectra of Co (top panels) and Ni (bottom panels) recorded on the CoTPP/Ni(001) system after the initial preparation of molecular adlayers (left), after NO addition (centre) and on temperature-induced NO desorption (right). The directions of the remanent substrate magnetization M are indicated by grey arrows to the left of each spectrum. Ferromagnetic ordering of molecular spins with respect to the substrate is observed initially. Reversible 'off–on' switching of Co magnetization is observed with progressing NO addition and temperature-induced NO desorption. Full size image XMCD spectroscopy X-ray absorption spectra of circularly polarized synchrotron light with opposite helicities (μ + and μ − ) are presented in Figure 1b . They clearly show a difference in absorption, that is, magnetic circular dichroism, at L 2 and L 3 absorption edges of both Co (top) and Ni (bottom). In the dichroic spectra, both the magnetic molecule (Co; Fig. 1c ; top left panel initial) and the substrate (Ni; Fig. 1c ; bottom left panel initial) show a magnetization, as characterized by the two peaks at photon energies corresponding to the L 2 and L 3 edges. A ferromagnetic coupling between CoTPP molecules and the Ni substrate is clearly identified by the same sign of the L 2 and L 3 dichroic signals in the respective spectra. Such ferromagnetic coupling has also been observed for similar molecules with different central metal atoms on various substrates [7] , [8] , [9] . Following numerical calculations based on density functional theory, this coupling occurs by superexchange through nitrogen atoms of the porphyrin ring for these observations [8] , [28] , [29] . To investigate the effect of a reaction with a chemical stimulus on the magnetization of CoTPP adsorbed on the Ni substrate, the CoTPP/Ni system was exposed to NO gas at room temperature. After the NO exposure, the initially well-detectable Co magnetization ( Fig. 1c ; initial) cannot be detected by XMCD anymore ( Fig. 1c ; '+NO). This behaviour is observed irrespective of the substrate magnetization and provides clear evidence that the magnetization of Co in CoTPP is switched off —an effect that goes far beyond earlier observations [7] , [8] , [21] and allows for the switching of individual molecular spins. As expected for a thin film, the Ni substrate magnetization was only marginally affected by the NO adsorption. We assign the off state of the molecular spin to the pairing of the initially unpaired Co spin, with the unpaired spin supplied by NO in the formation of a NO–CoTPP complex [22] , [23] , [30] as discussed further below. To probe the reversibility of the process the sample temperature was temporarily increased to ~615 K, leading to the removal of NO from the NO–CoTPP complex. This implies the reactivation of the Co spin ( S =½) and the regeneration of the ferromagnetic coupling between CoTPP and Ni as clearly reflected in the XMCD spectra ( Fig. 1c ; '−NO), that is, the Co spin system was switched on again. Consequently, the ferromagnetic coupling of Co magnetic moment to the Ni substrate magnetization is reestablished, as confirmed by the respective dichroic signals ( Fig. 1c ; '−NO). X-ray photoelectron spectroscopy To assess the influence of NO ligation on the chemical species involved and on the electronic interaction between CoTPP and Ni, we have employed X-ray photoelectron spectroscopy (XPS) and measured Co2p XP spectra at various stages of the experiment ( Fig. 2a ). For a monolayer of CoTPP on Ni, the Co2p 3/2 XPS signal exhibits a multiplet spectral feature, on which the main peak was observed at ~778.2 eV resembling an outermost ( d z 2 ) 1 -open-shell structure (compare CoTPP/Ag(111) system in Flechtner et al . [6] ). Reaction with NO causes two major changes in the Co2p 3/2 XPS signal. First, the multiplet spectral feature is replaced by a single peak, which is the expected behaviour for Co, assuming an outermost ( d z 2 ) 2 -closed-shell electronic structure. Second, the main peak position shifts from ~778.2 to ~780.2 eV—the latter value also being observed for the main Co2p 3/2 peak of CoTPP in multilayers (see Flechtner et al . [6] ). This behaviour suggests the suppression of the Co–Ni interaction by the stronger NO–Co interaction and correlates the observed chemical shift in XPS to a downshift of the unoccupied d z 2 spin level after bonding with NO. On thermal treatment of the NO–CoTPP–Ni system the multiplet feature of the Co2p 3/2 XPS signal, characterized by the main peak at ~778.2 eV, is observed again, which proves the NO dissociation from the nitrosyl complex—consistent with an earlier report on the electronic coupling of the NO–CoTPP–Ag system [6] . Notably, in our system, both the electronic coupling and the ad-molecular magnetization respond simultaneously to NO addition and removal. 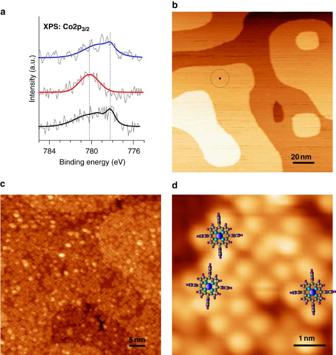Figure 2: Probing electronic interaction and visualizing molecules on the surface. (a) Co2p3/2XP spectra (raw data and fitted curves) of CoTPP molecules (~1 ML) on Ni(001) before NO exposure (black line), after NO exposure (red line) and on desorption of NO (blue line). The spectral evolution reflects the NO-induced reversible switching of the Co oxidation state and the modified electronic interaction between CoTPP molecules and the Ni surface. Different binding energy positions of the Co2p3/2XPS signal have been marked by dotted lines; 'a.u.' refers to arbitrary units. (b) Molecular adsorption on a reactive magnetic substrate: room temperature STM image showing the surface morphology of Ni(001) (150 nm × 150 nm; the size corresponding to one CoTPP molecule is depicted by the black square within the dotted circle). (c) Adsorption of CoTPP molecules on the Ni(001) surface (50 nm × 50 nm), where CoTPP is recognized by a four-leaf clover shape in symmetric and planar adsorption geometry while asymmetric conformations can also be detected38. (d) High-resolution STM: As a guide to the eye, molecular cartoons of CoTPP have been inserted (5 nm × 5 nm). Tunnelling parameters:I=0.07 nA,U=0.68 V (b) andI=0.05 nA,U=1.05 V (c,d). Figure 2: Probing electronic interaction and visualizing molecules on the surface. ( a ) Co2p 3/2 XP spectra (raw data and fitted curves) of CoTPP molecules (~1 ML) on Ni(001) before NO exposure (black line), after NO exposure (red line) and on desorption of NO (blue line). The spectral evolution reflects the NO-induced reversible switching of the Co oxidation state and the modified electronic interaction between CoTPP molecules and the Ni surface. Different binding energy positions of the Co2p 3/2 XPS signal have been marked by dotted lines; 'a.u.' refers to arbitrary units. ( b ) Molecular adsorption on a reactive magnetic substrate: room temperature STM image showing the surface morphology of Ni(001) (150 nm × 150 nm; the size corresponding to one CoTPP molecule is depicted by the black square within the dotted circle). ( c ) Adsorption of CoTPP molecules on the Ni(001) surface (50 nm × 50 nm), where CoTPP is recognized by a four-leaf clover shape in symmetric and planar adsorption geometry while asymmetric conformations can also be detected [38] . ( d ) High-resolution STM: As a guide to the eye, molecular cartoons of CoTPP have been inserted (5 nm × 5 nm). Tunnelling parameters: I =0.07 nA, U =0.68 V ( b ) and I =0.05 nA, U =1.05 V ( c , d ). Full size image Scanning tunnelling microscopy To further elucidate the nature of the chemical switching effect, it is necessary to study the adsorption geometry of the CoTPP molecules on Ni(001). Our scanning tunnelling microscopy (STM) data ( Fig. 2b–d ) show that the Ni(001) surface exhibits extended terraces that are virtually free of point defects and that CoTPP molecules adsorb spatially in a random distribution on the surface. This is due to a considerable surface-molecular interaction limiting the diffusion length during the deposition process, which then hinders the frequently observed self-assembly on metallic substrates [31] , [32] . This observation is in line with a recent report on the Mn-porphyrin/Co(001) system showing limited or no self-assembly [11] . High-resolution STM images of the CoTPP molecules on Ni(001) ( Fig. 2d ) reveal a planar orientation on the surface. A quasi-planar orientation has also been found by means of near-edge X-ray absorption fine structure spectroscopy for similar magnetic molecule–substrate interfaces, for example, Mn-porphyrin/Co(001), Fe-porphyrin/Co(001) and Fe-porphyrin/Ni(001) [7] , [8] . Density functional theory calculations have shown that magnetic exchange coupling requires the metalloporphyrin molecule: (i) in a planar orientation with the metal ion–4N moiety (see 'Co–4N' in Fig. 3a ) on the surface and (ii) in a certain distance from the magnetic substrate [8] , [28] , [29] . 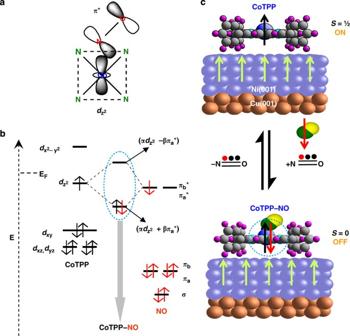Figure 3: Reversibleoff–onswitching of a molecular spin. (a) A scheme of the NO–CoTPP complex depicting the involvement of the relevant orbitals. The four green N atoms from the pyrrole moieties of the porphyrin represent the coordination with the Co ion and the dashed lines indicate the Co–4N plane that gets a pyramidal distortion on nitrosyl complex formation. (b) The electronic levels involved in the chemical reaction between NO acting as aπ-ligand and CoTPP. Molecular orbital diagrams (the dashed vertical arrow indicates the energy axis, E) of CoTPP (d7configuration: (dxz)2(dyz)2(dxy)2(dz2)1(dx2-y2)0adapted from Waylandet al.34and Kozuka and Nakamoto35) and NO (configuration: (σ)2(πa)2(πb)2(πa*)1(πb*)0adapted from Huheeyet al.23) showing the presence of unpaired electrons in both CoTPP (dz2) and NO (πa*). On formation of the NO–CoTPP complex (grey arrow), the unpaired spin of CoTPP, which is responsible for the molecular magnetism, is paired up with the unpaired spin supplied by NO in the mixed bonding orbital (highest occupied molecular orbital, HOMO). Consequently, the mixed antibonding orbital (lowest unoccupied molecular orbital, LUMO) is lifted above the Fermi level (EF) of the Ni substrate. Note that the energy levels of the orbitals within the blue dotted circle have been adapted from the literature: Waylandet al.34and Kozuka and Nakamoto35for the HOMO/LUMO of the NO–CoTPP complex and Flechtneret al.6for EF. α and β represent orbital mixing coefficients ofdz2andπa*, respectively. (c) Schematic representation of the switching process: switching on (top)—the CoTPP molecule is ferromagnetically coupled to the Ni substrate and the Co magnetic moment follows the substrate (Ni) magnetization; switchingoff(bottom)—on addition of NO, CoTPP (S=½) forms the NO–CoTPP complex (S=0) and the spin state of NO–CoTPP remains the same, irrespective of the Ni magnetization. Reversibility is shown by the reaction arrows indicating the chemical reaction with NO and the dissociation of NO. Figure 3: Reversible off–on switching of a molecular spin. ( a ) A scheme of the NO–CoTPP complex depicting the involvement of the relevant orbitals. The four green N atoms from the pyrrole moieties of the porphyrin represent the coordination with the Co ion and the dashed lines indicate the Co–4N plane that gets a pyramidal distortion on nitrosyl complex formation. ( b ) The electronic levels involved in the chemical reaction between NO acting as a π -ligand and CoTPP. Molecular orbital diagrams (the dashed vertical arrow indicates the energy axis, E) of CoTPP ( d 7 configuration: ( d xz ) 2 ( d yz ) 2 ( d xy ) 2 ( d z 2 ) 1 ( d x 2 - y 2 ) 0 adapted from Wayland et al . [34] and Kozuka and Nakamoto [35] ) and NO (configuration: (σ) 2 ( π a ) 2 ( π b ) 2 ( π a *) 1 ( π b *) 0 adapted from Huheey et al . [23] ) showing the presence of unpaired electrons in both CoTPP ( d z 2 ) and NO ( π a *). On formation of the NO–CoTPP complex (grey arrow), the unpaired spin of CoTPP, which is responsible for the molecular magnetism, is paired up with the unpaired spin supplied by NO in the mixed bonding orbital (highest occupied molecular orbital, HOMO). Consequently, the mixed antibonding orbital (lowest unoccupied molecular orbital, LUMO) is lifted above the Fermi level (E F ) of the Ni substrate. Note that the energy levels of the orbitals within the blue dotted circle have been adapted from the literature: Wayland et al . [34] and Kozuka and Nakamoto [35] for the HOMO/LUMO of the NO–CoTPP complex and Flechtner et al . [6] for E F . α and β represent orbital mixing coefficients of d z 2 and π a *, respectively. ( c ) Schematic representation of the switching process: switching on (top)—the CoTPP molecule is ferromagnetically coupled to the Ni substrate and the Co magnetic moment follows the substrate (Ni) magnetization; switching off (bottom)—on addition of NO, CoTPP ( S =½) forms the NO–CoTPP complex ( S =0) and the spin state of NO–CoTPP remains the same, irrespective of the Ni magnetization. Reversibility is shown by the reaction arrows indicating the chemical reaction with NO and the dissociation of NO. Full size image In our STM data, we observe some bright spots ( Fig. 2c ) that correspond to CoTPP molecules adsorbed on top of the first (incomplete) molecular layer. Molecules in the second layer do not have contact with the Ni substrate and reside comparably far above the surface. Thus, not every CoTPP molecule on our samples undergoes ferromagnetic exchange coupling with the Ni(001) substrate. However, XPS data ( Fig. 2a ) support that the vast majority of CoTPP molecules electronically interact with the Ni(001) substrate. Furthermore, in the STM overview of clean Ni(001) (cf. Fig. 2b ), the small black square drawn within the dotted circle represents the corresponding size of one CoTPP molecule. From the molecular dimensions and the step density observed in the STM data, we estimate an upper limit of ~5 to 10% of the molecules (at a coverage of ~1ML CoTPP), which can reside at low-symmetry sites, for example, step edges. As a result, most of the CoTPP molecules are adsorbed at high-symmetry sites and in planar orientation ( Fig. 2c and 2d ) and are thereby expected to contribute to the magnetic interaction and to respond well to the spin switching events by NO adsorption/desorption, as observed in the XMCD data (see Fig. 1c ). On the basis of the XPS identification of the Co species and the STM observation of a predominantly planar orientation of the molecules, the NO-induced reversible switching between CoTPP and Ni can be attributed to the trans effect [6] , [22] , [23] , [24] . In analogy to the elegant postulate reported in Flechtner et al . [6] describing the role of the trans effect in interfacial coordination chemistry, the NO ligand coordinating in trans position controls the coupling to a second ligand (Ni substrate) acting on the same metalloporphyrin (CoTPP). Bonding of NO with the Co ion presumably changes the 'Co–4N' planar geometry (see Fig. 3a ) such that the Co ion is pulled out of the plane towards the NO, whereby the overlap with Ni orbitals is reduced—which assists the switching event. The ' trans effect is frequently used to control chemical reactivity or electron affinity through ligands [22] , [23] , [24] and, as demonstrated here, simultaneously controls the chemical/electronic coupling and the spin state. The magnetic properties, namely the Co magnetization during the switching process that depends on the Ni substrate magnetization direction, can be uniquely probed for this system by the element-specific XMCD technique. The quenching of the Co XMCD signal observed in our experiments is identified as a consequence of the pairing of the originally unpaired spin in the d z 2 orbital on formation of the NO–CoTPP complex. This chemically stimulated process directly affects the Co spin system and the coupling to the substrate, as can be seen from the discussion of the molecular levels ( Fig. 3b ) involved: the highest occupied molecular orbital of the NO–CoTPP complex [33] , [34] , [35] originates from the interaction of singly occupied molecular orbitals of CoTPP ( d z 2 ) [34] , [35] and NO ( π *) [23] , as schematically shown in Figure 3a,b . On heating the sample, NO dissociates from the NO–CoTPP complex, leaving the CoTPP molecule with an unpaired spin and reestablishing the magnetoelectronic association with the Ni substrate. The dichroic signal at ~778.5 eV ( Fig. 1c ; top right panel) and the Co XPS data ( Fig. 2a ; blue line) clearly indicate that the CoTPP molecules remain intact after the temperature-induced dissociation of NO. A scheme for the NO-induced reversible switching of the magnetic response of CoTPP coupled to a ferromagnetic Ni substrate is presented in Figure 3c . Two different mechanisms can be considered: (i) NO reacts with CoTPP from the top and forms the NO–CoTPP complex or (ii) the Ni substrate reacts with NO and consequently affects the CoTPP–Ni interaction. To provide decisive evidence towards mechanism (i) or (ii), we have performed two additional experiments. First, a bare Ni(001) surface was exposed to ~6,000 L (Langmuir) of NO and was subsequently annealed at ~615 K. The O1s (a) and N1s (b) XPS signals (see Fig. 4 ) remain essentially unchanged on annealing. The shoulder observed at higher binding energies before annealing is assigned to physisorbed species desorbing from the surface on annealing. On the basis of the earlier reported observation of NO dissociation on Ni(001), even at room temperature [36] , the two peaks are attributed to Ni–N and Ni–O species, which remain chemisorbed at the annealing temperatures used in our experiment. 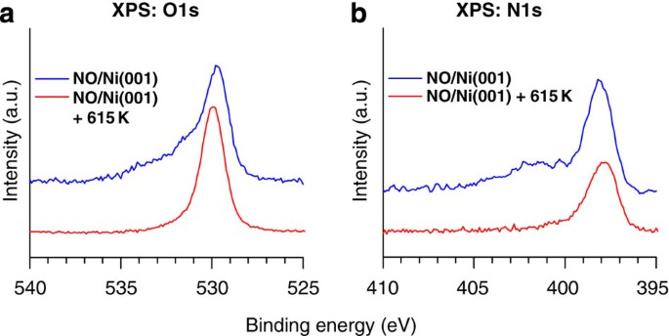Figure 4: Effect of NO coadsorption on Ni(001). XPS data recorded on a Ni(001) surface after exposure of ~6,000 L NO. The measurements were taken before (blue) and after (red) annealing at ~615 K. The O1s (a) and N1s (b) XP spectra clearly show that only the physisorbed NO is removed after annealing. The N/O intensity ratio is reduced after heating by a negligible extent, which suggests that the Ni(001) surface remained covered with nitrogen- and oxygen containing species even after annealing. We tentatively assign these species to chemisorbed Ni–oxygen/Ni–nitrogen and (NO)x. 'a.u.' represents arbitrary units. Figure 4: Effect of NO coadsorption on Ni(001). XPS data recorded on a Ni(001) surface after exposure of ~6,000 L NO. The measurements were taken before (blue) and after (red) annealing at ~615 K. The O1s ( a ) and N1s ( b ) XP spectra clearly show that only the physisorbed NO is removed after annealing. The N/O intensity ratio is reduced after heating by a negligible extent, which suggests that the Ni(001) surface remained covered with nitrogen- and oxygen containing species even after annealing. We tentatively assign these species to chemisorbed Ni–oxygen/Ni–nitrogen and (NO)x. 'a.u.' represents arbitrary units. Full size image In the second experiment, CoTPP (~1 ML) was deposited onto a Ni(001) surface preexposed to NO (~6,000 L). Subsequently, this system was annealed at ~615 K. Interestingly, the Co2p XPS data exhibited almost identical peak positions (Co2p 3/2 ~780.2 eV) before and after this annealing procedure (see Fig. 5 ), which indicates that CoTPP remains electronically decoupled from the Ni substrate, that is, the preexposure of NO modifies the Ni(001) substrate such that no NO-induced reversibility can be observed in this temperature window. These results confirm that our experiments on the NO-induced switching are not significantly determined/affected by side reactions of NO on the bare fraction of the Ni substrate (<20%; see Fig. 2b ), as the electronic and ferromagnetic exchange coupling between CoTPP and Ni is restored after annealing at ~615 K (see Figs 1c and 2a ). Thus, the reported experiments are all in agreement with mechanism (i) and are consistent with the involvement of the trans effect. Note that the observation of ligand-induced spin switching of porphyrins is not restricted to ferromagnetic substrates, and we expect that this work can be extended to antiferromagnetic or diamagnetic (for example, Cu(100)) substrates as well, using sufficiently high external magnetic fields at low temperature, for example, 6 T and 8 K [21] . The trans effect, as used to control the site-specific affinity of porphyrins or phthalocyanines to chemical reactants, is used in this study to control the spin localized at a central metal ion, and thereby provides the case for a spin trans effect. 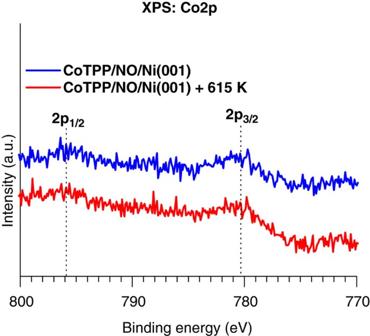Figure 5: Role of thetranseffect in the observed reversibility. About 1 ML of CoTPP was evaporated onto a Ni(001) surface that was previously exposed to ~6,000 L of NO to prepare a CoTPP/NO/Ni(001) system. The system was subsequently annealed at ~615 K, and Co2p XP spectra were recorded before and after annealing. Before annealing, the Co2p3/2peak at ~780.2 eV indicates that there is no electronic interaction between CoTPP and Ni. Interestingly, even after annealing, the CoTPP remained electronically decoupled from the Ni. This control experiment shows that CoTPP on preexposed NO/Ni(001) cannot exhibit reversibility of the magnetoelectronic interaction between CoTPP and Ni (seeFigs 1cand2a). Thereby, the reversibility observed in our main experiment is attributed to gaseous NO species coordinating to the CoTPP adlayer through thetranseffect6. 'a.u.' represents arbitrary units. Figure 5: Role of the trans effect in the observed reversibility. About 1 ML of CoTPP was evaporated onto a Ni(001) surface that was previously exposed to ~6,000 L of NO to prepare a CoTPP/NO/Ni(001) system. The system was subsequently annealed at ~615 K, and Co2p XP spectra were recorded before and after annealing. Before annealing, the Co2p 3/2 peak at ~780.2 eV indicates that there is no electronic interaction between CoTPP and Ni. Interestingly, even after annealing, the CoTPP remained electronically decoupled from the Ni. This control experiment shows that CoTPP on preexposed NO/Ni(001) cannot exhibit reversibility of the magnetoelectronic interaction between CoTPP and Ni (see Figs 1c and 2a ). Thereby, the reversibility observed in our main experiment is attributed to gaseous NO species coordinating to the CoTPP adlayer through the trans effect [6] . 'a.u.' represents arbitrary units. Full size image Because of the large body of knowledge about porphyrins and phthalocyanines [1] , and their variability established in coordination chemistry, the spin trans effect is expected to proceed beyond the case presented here. Spin switching systems on the basis of the presented architecture are expected to be demonstrated using other chemical stimuli (for example, CO), using modified molecular spin systems (for example, metallophthalocyanines), and also for the case of antiferromagnetic exchange coupling [10] , [11] . Considering the involvement of the chromophoric group in these molecules, the use of other stimuli such as light is foreseeable. By exploiting a pump-and-probe approach it might become possible to study spin dynamics in surface-supported chemical reactions using the XMCD technique [20] . The reversible off–on switching of the electron spin in a surface-supported paramagnetic molecule presented here suggests further studies on organic spintronic interfaces in conjunction with transport measurements. In view of the rapidly advancing capabilities to induce events on the level of single atoms and molecules by scanning probe microscopy, it is anticipated that surface-supported magnetic molecules can be individually switched. The behaviour of such model systems, not only as isolated spin systems and in dependence of their coupling to the substrate/environment but also as elements of quantum-coupled systems, may provide a new basis for experimental insight into quantum behaviour at further increased complexity. Sample preparation and characterization All experiments were performed in ultrahigh vacuum. Cu(001) single crystals (MaTecK GmbH) were cleaned by repeated Ar + sputtering/annealing cycles and the impurity level was monitored by recording C1s, O1s, N1s and Ni2p XPS signals. Ni (MaTecK GmbH) thin films (~20 MLs, ~3.5 nm) were deposited by means of electron-beam evaporation in a two-step procedure onto clean Cu(001) single crystals [11] . In the first step, ~10 MLs of Ni were evaporated on Cu(001) kept at room temperature, which provided a sufficient barrier to prevent the Cu atoms from diffusion across the Ni layers. After ~30 min of annealing at ~530 K, another ~10 MLs of Ni were deposited while keeping the sample at ~460 K to obtain atomically flat terraces. During these evaporation steps, the deposition rate was monitored by a quartz crystal microbalance. After deposition of ~20 MLs of Ni on Cu(001), the thin-film substrate was investigated by XPS and low-energy electron diffraction studies to assure that no contamination of the film occurred and that the growing film shows the fcc(001) structure [11] . CoTPP (Sigma-Aldrich) molecules were evaporated (~1 ML) onto a freshly prepared non-magnetized Ni(001) substrate kept at room temperature. The deposition rate was monitored by a quartz crystal microbalance and the molecular coverage on the surface was calibrated by combined XPS and STM measurements. STM images were taken in constant-current mode at room temperature with a Pt/Ir tip and the bias voltages were referred to the grounded sample. The prepared samples were transported to the surfaces/interfaces microscopy (SIM) beamline of the Swiss Light Source (SLS) using a vacuum suitcase (base pressure in the order of ~7.5×10 −11 Torr), that is, without breaking the vacuum. XMCD measurements An external magnetic field of ~125 mT was applied perpendicular to the surface plane of the CoTPP/Ni(001) sample before the XMCD measurements to assure single-domain magnetization of the Ni film along the easy axis (out-of-plane) [8] . The L-edges absorption spectra for both Co and Ni were recorded at normal incidence in total electron yield mode without externally applied magnetic field, that is, in the remanent magnetization of the Ni substrate. The SLS-SIM beamline provides high brilliance X-ray light in the energy range of 130–2,000 eV from two elliptical twin undulators, which permit switching of the photon helicity optically within a few seconds [37] . All spectra were recorded at room temperature and normalized to the incident photon flux. The Ni magnetization was reproducibly reversed by inverting the externally applied magnetic field. XMCD data taken at the SLS-SIM beamline were complemented by XPS/STM measurements using the same sample preparation conditions. NO dosing and heating The CoTPP/Ni(001) system was exposed to ~6,000 L of NO (exposure time ~17 min) in the XMCD chamber at room temperature. The sample was subsequently heated to ~615 K to remove NO from the NO–CoTPP complex. Notably, our experiments suggest that cooling the sample to ~100 K reduces the required NO exposure to a considerable extent, whereas the off–on electronic switching events can still be consistently observed by the XPS measurements. How to cite this article : Wäckerlin, C. et al . Controlling spins in adsorbed molecules by a chemical switch. Nat. Commun. 1:61 doi: 10.1038/ncomms1057 (2010).